The small-molecule BGP-15 protects against heart failure and atrial fibrillation in mice Heart failure (HF) and atrial fibrillation (AF) share common risk factors, frequently coexist and are associated with high mortality. Treatment of HF with AF represents a major unmet need. Here we show that a small molecule, BGP-15, improves cardiac function and reduces arrhythmic episodes in two independent mouse models, which progressively develop HF and AF. In these models, BGP-15 treatment is associated with increased phosphorylation of the insulin-like growth factor 1 receptor (IGF1R), which is depressed in atrial tissue samples from patients with AF. Cardiac-specific IGF1R transgenic overexpression in mice with HF and AF recapitulates the protection observed with BGP-15. We further demonstrate that BGP-15 and IGF1R can provide protection independent of phosphoinositide 3-kinase-Akt and heat-shock protein 70; signalling mediators often defective in the aged and diseased heart. As BGP-15 is safe and well tolerated in humans, this study uncovers a potential therapeutic approach for HF and AF. With a growing ageing population and increased incidence of obesity and diabetes, the prevalence of heart failure (HF) and atrial fibrillation (AF; the most common sustained cardiac arrhythmia) is rising [1] , [2] . HF and AF frequently coexist because they share common risk factors, have overlapping underlying pathologies, and each condition predisposes to the other [3] . Individually, HF and AF are associated with significant morbidity and mortality, and the presence of both identifies patients with a higher risk of death than either condition alone [2] , [4] . Current drugs have limited or no efficacy, and potentially dangerous side effects [5] , [6] , [7] . Thus, the treatment of patients with HF and AF represents a major unmet need [7] , [8] . The major goal of the current study was to assess the therapeutic potential of a small molecule, a hydroximic acid derivative named BGP-15, in a mouse model, which develops HF and is susceptible to AF. BGP-15 is administered orally and has been shown to have an excellent safety profile in multiple human clinical trials in healthy individuals [9] , [10] and insulin-resistant non-diabetic patients [11] . The initial rationale for assessing the therapeutic potential of BGP-15 in an animal model with a failing heart and increased susceptibility to AF was related to its role as a co-inducer of the stress inducible form of heat-shock protein 70 (HSP70/72) [12] . Studies in animal models and/or humans suggested that elevated levels of HSP70 (endogenous, genetically manipulated, drug-induced or hyperthermia-induced) were protective against the development of AF, and/or cardiac pathology in settings of ischaemia [13] , [14] , [15] , [16] , [17] , [18] . Furthermore, reduced/defective cardiac HSP70 was associated with an increased risk of postoperative AF in humans [15] , [16] . Here we show that BGP-15 can reduce episodes of arrhythmia, attenuate atrial enlargement and improve cardiac function in two different murine models with HF and AF. Contrary to our initial hypothesis, however, the mechanism of action was not via induction of HSP70. Instead, BGP-15 treatment was associated with increased phosphorylation of the insulin-like growth factor 1 receptor (pIGF1R; IGF1R is a key protective factor in the heart [19] ). As BGP-15 is safe in humans, this drug offers a possible therapeutic approach for HF and AF patients. BGP-15 improves cardiac function in a HF+AF mouse model We previously described a transgenic (Tg) mouse model with a failing heart, which is susceptible to AF (referred to here as HF+AF model) [20] . In brief, the model was generated by breeding a cardiac-specific Tg mouse with a failing heart because of dilated cardiomyopathy (DCM, induced with increased activity of mammalian sterile 20-like kinase 1, Mst1; a kinase activated by clinically important pathologic insults such as ischaemia/reperfusion [21] ) with a cardiac-specific Tg mouse with reduced phosphoinositide 3-kinase (PI3K; because of expression of a dominant negative PI3K (dnPI3K) mutant [22] ). Risk factors for HF and AF, including ageing, obesity and diabetes, have been associated with insulin resistance that can lead to depressed/defective PI3K signalling [23] , [24] , [25] , and PI3K activity was also depressed in atrial tissue from patients with AF [20] . Reducing PI3K in the mouse model with DCM accelerated the HF phenotype based on the following findings: additional systolic dysfunction, substantial atrial enlargement, increased fibrosis and elevated lung weights [20] . At 4 months of age, the HF+AF model was also associated with electrocardiogram (ECG) abnormalities including intermittent/episodic AF (irregular heart rhythm with loss of P waves confirmed by intracardiac ECG recordings) [20] . A feature of HF and AF in humans and animal models is electrical remodelling, typically associated with mutations or changes in expression of ion channels and connexins [26] . The functional significance of these changes are not completely understood, and the regulation (up or down) of channels and/or connexins may vary depending on the species, duration and/or model of HF and AF [26] , [27] . It is noteworthy, however, that a number of channels and connexins are also differentially regulated in cardiac tissue of the HF+AF mouse model ( Supplementary Fig. 1, for example, Scn5a , Kcna5 and Gja5 /Cx40). Finally, consistent with the incidence of HF and AF increasing with age in humans, the phenotype of the HF+AF mouse model also gets progressively worse with age based on cardiac morphology, function and ECG parameters ( Supplementary Fig. 2 : comparison at 5 and 8 months of age). Adult (~4 month) male HF+AF and non-Tg (Ntg) littermates were administered with BGP-15 (15 mg kg −1 per day in saline) for 4 weeks by oral gavage or remained untreated (oral gavage with saline or no gavage). Gavage with saline had no effect on morphological parameters or cardiac dimensions in the HF+AF model ( Supplementary Fig. 3 ). Thus, untreated mice (no gavage) and mice administered saline have been combined and referred to as HF+AF control. Cardiac function (assessed by echocardiography) and ECG studies were performed before and after treatment. BGP-15 treatment had no effect in Ntg mice or an independent cohort of normal adult wild-type mice based on morphology, cardiac function and ECG parameters ( Supplementary Tables 1–6 , Supplementary Figs 4,5 ). The HF+AF model is associated with significant atrial enlargement ( Fig. 1a,b ), lung congestion ( Fig. 1c ) and cardiac dysfunction (fractional shortening in HF+AF~25% versus Ntg~48%; Supplementary Table 2 ). 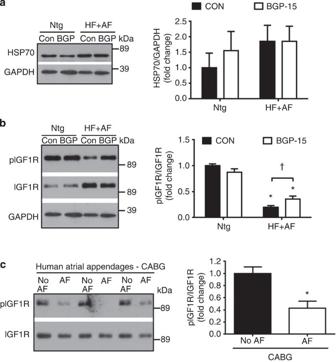Figure 2: pIGF1R is decreased in atrial tissue from the HF+AF model and patients with AF, and increased with BGP-15 treatment. (a,b) Western blots and quantification of HSP70 relative to GAPDH and pIGF1R relative to total IGF1R in mouse atria. *P<0.05 versus Ntg control (CON) and Ntg BGP-15;†P<0.05 versus HF+AF CON.N=4–5 per group. Data are mean±s.e.m.Pvalues calculated by one-way analysis of variance followed by Fisher least significant differencepost hocpairwise test. (c) Western blots and quantification of pIGF1R relative to total IGF1R in atrial samples from patients undergoing CABG who did or did not develop AF. Data are mean±s.e.m. *P<0.05 versus CABG with no AF.N=4 per group (unpairedt-test). GAPDH, glyceraldehyde 3-phosphate dehydrogenase. 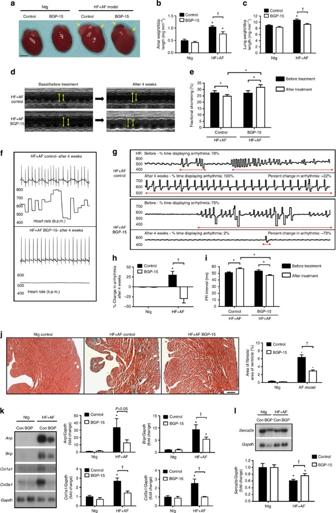Treatment with BGP-15 attenuated the increase in atrial size and lung weight ( Fig. Figure 1: BGP-15 attenuates cardiac pathology, improves cardiac function and reduces episodes of arrhythmia in the HF+AF model. (a) Representative heart photos from control and BGP-15-treated Ntg and HF+AF mice. Yellow arrows highlight the smaller atrial size in BGP-15-treated HF+AF mice versus HF+AF control mice. Scale bar, 2.5 mm. (b,c) Quantification of atria weight/tibia length and lung weight/tibia length. *P<0.05 versus Ntg control and Ntg BGP-15;†P<0.05.N=4–6 for Ntg groups and 7–15 for HF+AF groups. (d) Representative M-mode echocardiograms from control and BGP-15-treated HF+AF mice before and after treatment. Yellow arrows highlight differences in LV chamber dimensions. (e) Quantification of fractional shortening before and after treatment. *P<0.05,N=7 per group. (f) Representative ECG traces (upper panel) and heart rate (HR) variability (lower panel) in the HF+AF model after 4 weeks±BGP-15. (g) HR recordings (b.p.m.) from HF+AF control and BGP-15-treated HF+AF mice (Areas of arrhythmia are highlighted with red arrows. To be considered non-arrhythmic, the HR had to be stable for >4 s. Each trace represents 20 s.), and (h) quantification of the % change in arrhythmia after 4 weeks. *P<0.05 versus Ntg control and Ntg BGP-15;†P<0.05.N=4–6 for Ntg groups and 7–13 for HF+AF groups. (i) Quantification of PR intervals before and after treatment. *P<0.05N=7–13 per group. (j) LV cross-sections stained with Masson’s trichrome (fibrosis stains blue, magnification × 40; scale bar, 200 μm) and quantification (right panel).N=3–4 for Ntg groups and 5–6 for HF+AF groups. Visually and quantitatively BGP-15 had no effect in Ntg mice. (k,l) Northern blots and quantification ofAnp,Bnp,Col1a1,Col3a1andSerca2arelative toGapdh.N=3–4 for Ntg groups and 5–8 for HF+AF groups. *P<0.05 versus Ntg control and Ntg BGP-15;†P<0.05. Data are mean±s.e.m. Forb,c,e,h–l,Pvalues calculated by one-way analysis of variance followed by Fisher least significant differencepost hocpairwise test. Foreandi,Pvalues calculated by pairedt-test when comparing the same mice before and after treatment. 1a–c , Supplementary Table 1 ), and this was associated with improved cardiac function (left ventricular (LV) dimensions and systolic function, Fig. 1d,e , Supplementary Table 2 ). Control HF+AF mice displayed increased episodes of arrhythmia over the 4-week study period ( Fig. 1f–h ). In contrast, BGP-15 treatment was able to prevent or reduce episodes of arrhythmia ( Fig. 1f–h ). As the HF+AF mouse model displays episodic AF, PR interval was used as an additional marker of disease status. Prolonged PR intervals in disease settings have been associated with AF, HF and death in humans [28] , [29] , [30] . Consistent with this association, PR interval deteriorates in the HF+AF model with age and disease progression ( Supplementary Fig. 2 ). BGP-15 treatment was associated with a reduced PR interval in the HF+AF model ( Fig. 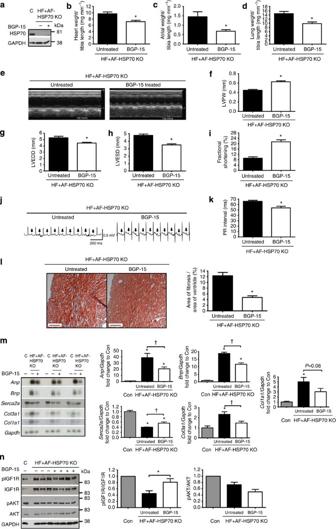Figure 3: BGP-15 mediates protection in the HF+AF model independently of HSP70. (a) Western blot showing HSP70 is deleted in ventricles of HF+AF-HSP70 KO mice. (b–d) Quantification of heart weight, atria weight and lung weight relative to tibia length.N=5 per group. (e) Representative M-mode echocardiograms of untreated and BGP-15-treated HF+AF-HSP70 KO mice. (f–i) Left ventricular (LV) posterior wall thickness (LVPW), LV end-diastolic dimension (LVEDD), LV end systolic dimension (LVESD) and fractional shortening.N=4–5 per group. (j) ECG traces of an untreated and BGP-15-treated HF+AF-HSP70 KO mouse. Arrows signify P waves. (k) PR interval.N=4–5 per group. (l) LV cross-sections stained with Masson’s trichrome (magnification × 40; scale bar, 200 μm) and quantification of fibrosis.N=3 per group.b–d,f–i,k–l: *P<0.05 versus untreated HF+AF-HSP70 KO. (m) Northern blots and quantification ofAnp,Bnp,Serca2a, Col3a1andCol1a1relative toGapdh.N=3–4 per group. *P<0.05 versus control;†P<0.05. (n) Western blots and quantification of pIGF1R relative to IGF1R and pAkt relative to total Akt in mouse ventricle. *P<0.05.N=5 per group for HF+AF-HSP70 KO. Control (Con, C) represents RNA or protein from heart(s) of Ntg mice to highlight changes with the HF+AF-HSP70 KO model. Data are mean±s.e.m. Forb–d,f–i,k–l,nPvalues calculated by unpairedt-test; (m)Pvalues calculated by one-way analysis of variance followed by Fisher least significant differencepost hocpairwise test. GAPDH, glyceraldehyde 3-phosphate dehydrogenase. 1i , Supplementary Table 3 ). Figure 1: BGP-15 attenuates cardiac pathology, improves cardiac function and reduces episodes of arrhythmia in the HF+AF model. ( a ) Representative heart photos from control and BGP-15-treated Ntg and HF+AF mice. Yellow arrows highlight the smaller atrial size in BGP-15-treated HF+AF mice versus HF+AF control mice. Scale bar, 2.5 mm. ( b , c ) Quantification of atria weight/tibia length and lung weight/tibia length. * P <0.05 versus Ntg control and Ntg BGP-15; † P <0.05. N =4–6 for Ntg groups and 7–15 for HF+AF groups. ( d ) Representative M-mode echocardiograms from control and BGP-15-treated HF+AF mice before and after treatment. Yellow arrows highlight differences in LV chamber dimensions. ( e ) Quantification of fractional shortening before and after treatment. * P <0.05, N =7 per group. ( f ) Representative ECG traces (upper panel) and heart rate (HR) variability (lower panel) in the HF+AF model after 4 weeks±BGP-15. ( g ) HR recordings (b.p.m.) from HF+AF control and BGP-15-treated HF+AF mice (Areas of arrhythmia are highlighted with red arrows. To be considered non-arrhythmic, the HR had to be stable for >4 s. Each trace represents 20 s.), and ( h ) quantification of the % change in arrhythmia after 4 weeks. * P <0.05 versus Ntg control and Ntg BGP-15; † P <0.05. N =4–6 for Ntg groups and 7–13 for HF+AF groups. ( i ) Quantification of PR intervals before and after treatment. * P <0.05 N =7–13 per group. ( j ) LV cross-sections stained with Masson’s trichrome (fibrosis stains blue, magnification × 40; scale bar, 200 μm) and quantification (right panel). N =3–4 for Ntg groups and 5–6 for HF+AF groups. Visually and quantitatively BGP-15 had no effect in Ntg mice. ( k , l ) Northern blots and quantification of Anp , Bnp , Col1a1 , Col3a1 and Serca2a relative to Gapdh . N =3–4 for Ntg groups and 5–8 for HF+AF groups. * P <0.05 versus Ntg control and Ntg BGP-15; † P <0.05. Data are mean±s.e.m. For b , c , e , h – l , P values calculated by one-way analysis of variance followed by Fisher least significant difference post hoc pairwise test. For e and i , P values calculated by paired t -test when comparing the same mice before and after treatment. Full size image Cardiac fibrosis and molecular markers associated with cardiac pathology (atrial and B-type natriuretic peptides ( Anp and Bnp )) and collagen deposition (collagen 1 ( Col1a1 ) and collagen 3 ( Col3a1 )) were elevated in the hearts of the HF+AF control model (versus Ntg) but were attenuated by BGP-15 ( Fig. 1j,k ). Furthermore, sarcoplasmic/endoplasmic reticulum Ca 2+ -ATPase 2a ( Serca2a ) gene expression, known to be important for maintaining cardiac contractility, was higher in hearts of the BGP-15-treated HF+AF model compared with HF+AF control ( Fig. 1l ). BGP-15 increases pIGF1R, which is lower in mouse and human AF Based on the known role of BGP-15 as a HSP coinducer, and previous studies demonstrating an increase in HSP70 in other muscles of BGP-15-treated mice (skeletal and diaphragm) [31] , [32] , we had hypothesized the protection provided by BGP-15 would be associated, at least in part, with an increase in HSP70 in cardiac tissue. Contrary to this, we observed no increase in HSP70 in atrial tissue from BGP-15-treated mice ( Fig. 2a ). We also examined the expression of another HSP previously associated with AF, HSP27 (ref. 33 ). HSP27 was elevated in the HF+AF model, but remained unchanged with BGP-15 treatment ( Supplementary Fig. 6 ). Figure 2: pIGF1R is decreased in atrial tissue from the HF+AF model and patients with AF, and increased with BGP-15 treatment. ( a , b ) Western blots and quantification of HSP70 relative to GAPDH and pIGF1R relative to total IGF1R in mouse atria. * P <0.05 versus Ntg control (CON) and Ntg BGP-15; † P <0.05 versus HF+AF CON. N =4–5 per group. Data are mean±s.e.m. P values calculated by one-way analysis of variance followed by Fisher least significant difference post hoc pairwise test. ( c ) Western blots and quantification of pIGF1R relative to total IGF1R in atrial samples from patients undergoing CABG who did or did not develop AF. Data are mean±s.e.m. * P <0.05 versus CABG with no AF. N =4 per group (unpaired t -test). GAPDH, glyceraldehyde 3-phosphate dehydrogenase. Full size image In addition to acting as a HSP-coinducer, BGP-15 has also been shown to enhance the actions of membrane-localized receptor proteins, including the insulin receptor [12] , [34] . Accordingly, we next assessed the phosphorylation of the IGF1R, an insulin receptor family member known to mediate protection in the heart [19] . The phosphorylation of IGF1R relative to total IGF1R was depressed in atrial tissue from the HF+AF control model compared with Ntg, and this was higher in HF+AF mice treated with BGP-15 ( Fig. 2b ). To ascertain whether IGF1R may play a role in the pathogenesis of AF in humans, we assessed phosphorylation of IGF1R in atrial appendages from age-matched patients who had undergone coronary artery bypass graft (CABG) surgery, who did or did not develop AF postoperatively (patient characteristics presented in Supplementary Table 7 ) [20] . Phosphorylation of IGF1R was approximately 60% lower in atrial appendages from patients with AF compared with samples from those who remained in sinus rhythm ( Fig. 2c ). 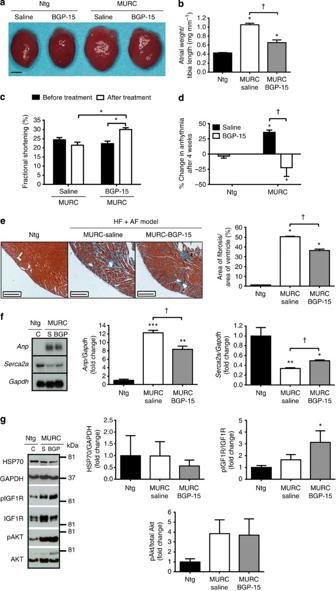Figure 7: BGP-15 attenuates cardiac pathology and episodes of arrhythmia, and improves cardiac function in the MURC model. (a) Representative heart photos from saline and BGP-15-treated Ntg and MURC mice. Scale bar, 2.5 mm. (b) Quantification of atria weight/tibia length. *P<0.05 versus Ntg control;†P<0.05.N=3 for Ntg control and 4 for MURC groups. (c) Quantification of fractional shortening before and after treatment. *P<0.05,N=4 per group. (d) Quantification of the % change in arrhythmia after 4 weeks. *P<0.05 versus Ntg control;†P<0.05.N=3 for Ntg control and 4 for MURC groups. (e) LV cross-sections stained with Masson’s trichrome (fibrosis stains blue, magnification × 40; scale bar, 400 μm) and quantification (right panel). *P<0.05 versus Ntg control;†P<0.05.N=3 for Ntg control and 4 for MURC groups. (f) Northern blots and quantification ofAnpandSerca2arelative toGapdh.N=3 for Ntg control and 4 for MURC groups. *P<0.05 versus Ntg control; **P<0.005, ***P<0.001 versus Ntg control;†P<0.05. (g) Western blots and quantification of HSP70 relative to GAPDH, pIGF1R relative to total IGF1R and pAkt relative to total Akt in mouse atria. *P<0.05 versus Ntg control.N=3 for Ntg control and 4 for MURC groups. Data are mean±s.e.m. Forb,d–g,Pvalues calculated by one-way analysis of variance followed by Fisher least significant differencepost hocpairwise test. Forc,Pvalues calculated by pairedt-test when comparing the same mice before and after treatment, or one-way analysis of variance followed by Fisher least significant differencepost hocpairwise test. BGP-15 is protective in HF+AF mice independently of HSP70 HSP70 protein expression data obtained from the HF+AF model administered BGP-15 suggested that HSP70 was not contributing to the cardiac protection observed ( Fig. 2a ). However, activation of signalling mediators can be transient, and previous studies in other tissues demonstrated BGP-15 was able to induce HSP70 (refs 31 , 32 ). To definitively assess the role of HSP70 in our experimental model, two additional mouse models were generated and characterized. First, we generated the HF+AF model with HSP70 deleted (that is, HF+AF-HSP70 knockout, KO) and administered BGP-15 (15 mg kg −1 per day, oral gavage) for 4 weeks. Second, we generated mice in which HSP70 was overexpressed in the hearts of the HF+AF model using a Tg approach (that is, HF+AF-HSP70 Tg). BGP-15 was able to mediate protection in mice in which HSP70 had been deleted, that is, HF+AF-HSP70 KO mice ( Fig. 3a ) based on multiple parameters including morphology ( Fig. 3b–d , Supplementary Table 8 ), LV dimensions and function ( Fig. 3e–i , Supplementary Table 9 ), ECG parameters ( Fig. 3j,k , Supplementary Table 10 ), cardiac fibrosis ( Fig. 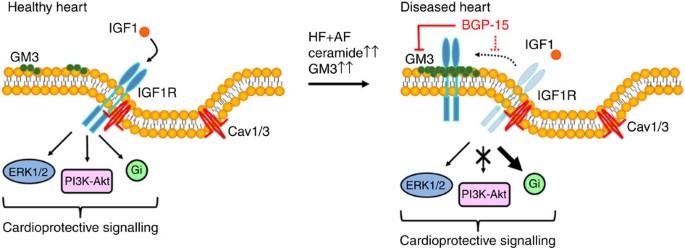Figure 8: Schematic representation of BGP-15 protection in a setting of HF and AF. We propose that binding of IGF1R with caveolin-1 and caveolin-3 is important for IGF1R-protective signalling. In the HF+AF model, ganglioside GM3 levels are increased and this disrupts the interaction between IGF1R and caveolins. BGP-15 can restore signalling by attenuating GM3 levels. In the diseased setting, the dotted black line shows the proposed disruption of IGF1R with caveolins because of increased GM3. BGP-15 attenuated GM3 (solid red line) and may attenuate the dissociation between IGF1R and caveolins (dotted red line). In the HF+AF model, PI3K-Akt signalling is blunted (as indicated with a cross, X). The current results suggest IGF1R may mediate protection via Gi, although this will require further investigation. 3l ) and molecular markers ( Anp , Bnp , Serca2a , Col3a1 , Col1a1 ; Fig. 3m ). BGP-15 treatment was also associated with increased phosphorylation of IGF1R in cardiac tissue from HF+AF-HSP70 KO mice; without an increase in the phosphorylation of Akt ( Fig. 3n ). Finally, increasing HSP70 expression in the HF+AF model ( Supplementary Fig. 7a ) conveyed no benefit based on morphology, histology or molecular markers ( Supplementary Fig. 7b–e , Supplementary Table 11 ). Figure 3: BGP-15 mediates protection in the HF+AF model independently of HSP70. ( a ) Western blot showing HSP70 is deleted in ventricles of HF+AF-HSP70 KO mice. ( b – d ) Quantification of heart weight, atria weight and lung weight relative to tibia length. N =5 per group. ( e ) Representative M-mode echocardiograms of untreated and BGP-15-treated HF+AF-HSP70 KO mice. ( f – i ) Left ventricular (LV) posterior wall thickness (LVPW), LV end-diastolic dimension (LVEDD), LV end systolic dimension (LVESD) and fractional shortening. N =4–5 per group. ( j ) ECG traces of an untreated and BGP-15-treated HF+AF-HSP70 KO mouse. Arrows signify P waves. ( k ) PR interval. N =4–5 per group. ( l ) LV cross-sections stained with Masson’s trichrome (magnification × 40; scale bar, 200 μm) and quantification of fibrosis. N =3 per group. b – d , f – i , k – l : * P <0.05 versus untreated HF+AF-HSP70 KO. ( m ) Northern blots and quantification of Anp , Bnp , Serca2a, Col3a1 and Col1a1 relative to Gapdh . N =3–4 per group. * P <0.05 versus control; † P <0.05. ( n ) Western blots and quantification of pIGF1R relative to IGF1R and pAkt relative to total Akt in mouse ventricle. * P <0.05. N =5 per group for HF+AF-HSP70 KO. Control (Con, C) represents RNA or protein from heart(s) of Ntg mice to highlight changes with the HF+AF-HSP70 KO model. Data are mean±s.e.m. For b – d , f – i , k – l , n P values calculated by unpaired t -test; ( m ) P values calculated by one-way analysis of variance followed by Fisher least significant difference post hoc pairwise test. GAPDH, glyceraldehyde 3-phosphate dehydrogenase. Full size image Increased IGF1R is reminiscent of BGP-15-mediated protection To examine whether the increased activation of IGF1R in hearts of BGP-15-treated HF+AF mice ( Fig. 2b ) played a significant role in providing protection, HF+AF mice overexpressing IGF1R specifically in cardiac myocytes (HF+AF-IGF1R Tg) were generated and characterized at approximately 4 months of age. This was of particular interest because the cardioprotective properties of IGF1R have largely been attributed to activation of PI3K, which is significantly blunted in the HF+AF model because of incorporation of the dnPI3K transgene [20] , [22] . First, increased expression of IGF1R in cardiac tissue of HF+AF-IGF1R Tg mice was confirmed ( Fig. 4a ), and this occurred in the absence of an increase in the phosphorylation of Akt (downstream target of PI3K, Fig. 4a ). Tg expression of IGF1R alone induced physiological cardiac hypertrophy, characterized by increased cardiac tissue weights and improved systolic function ( Fig. 4b–i see IGF1R), as previously reported [19] . HF+AF-IGF1R Tg displayed more favourable morphological features compared with the HF+AF model alone, most notably an attenuation of lung congestion and a trend for reduced atrial weight ( Fig. 4c,d , Supplementary Table 12 ). HF+AF-IGF1R Tg also showed more favourable LV dimensions and improved systolic function compared with the HF+AF model alone ( Fig. 4e–i , Supplementary Table 13 ), more regular ECG traces and reduced PR intervals ( Fig. 4j,k , Supplementary Table 14 ). IGF1R-induced protection was associated with less cardiac fibrosis ( Fig. 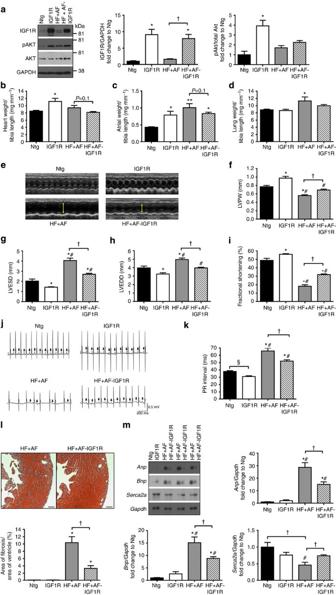4l ), lower Anp and Bnp expression, and higher Serca2a gene expression ( Fig. 4m ). Figure 4: Transgenic overexpression of IGF1R in the HF+AF mouse model resembles BGP-15-mediated protection. (a) Representative western blots and quantification of IGF1R relative to GAPDH and pAkt relative to total Akt.N=3–6 per group. (b–d) Graphs of heart weight/tibia length (TL), atria weight/TL and lung weight/TL.N=4–7 per group. (e) M-mode echocardiograms of Ntg, IGF1R, HF+AF and HF+AF-IGF1R mice. Yellow arrows highlight differences in left ventricular (LV) dimensions. (f–i) LV posterior wall thickness (LVPW), LV end systolic dimension (LVESD), LV end-diastolic dimension (LVEDD) and fractional shortening.N=3–6 per group. (j) ECG traces of Ntg, IGF1R, HF+AF and HF+AF-IGF1R mice. Arrows signify P waves. (k) PR interval.N=3–6 per group. (l) LV cross-sections stained with Masson’s trichrome (magnification × 40; scale bar, 200 μm) and quantification of fibrosis (lower panel).N=4–7 per group. (m) Northern blots and quantification ofAnp,BnpandSerca2arelative toGapdh.N=4–6 per group. Data are mean±s.e.m. Fora–d,f–i,k–m, *P<0.05 versus Ntg, **P<0.01 versus Ntg,#P<0.05 versus IGF1R,†P<0.05.Pvalues calculated by one-way analysis of variance followed by Fisher least significant differencepost hocpairwise test. Fork,§P<0.05 versus Ntg (unpairedttest). GAPDH, glyceraldehyde 3-phosphate dehydrogenase. Figure 4: Transgenic overexpression of IGF1R in the HF+AF mouse model resembles BGP-15-mediated protection. ( a ) Representative western blots and quantification of IGF1R relative to GAPDH and pAkt relative to total Akt. N =3–6 per group. ( b – d ) Graphs of heart weight/tibia length (TL), atria weight/TL and lung weight/TL. N =4–7 per group. ( e ) M-mode echocardiograms of Ntg, IGF1R, HF+AF and HF+AF-IGF1R mice. Yellow arrows highlight differences in left ventricular (LV) dimensions. ( f – i ) LV posterior wall thickness (LVPW), LV end systolic dimension (LVESD), LV end-diastolic dimension (LVEDD) and fractional shortening. N =3–6 per group. ( j ) ECG traces of Ntg, IGF1R, HF+AF and HF+AF-IGF1R mice. Arrows signify P waves. ( k ) PR interval. N =3–6 per group. ( l ) LV cross-sections stained with Masson’s trichrome (magnification × 40; scale bar, 200 μm) and quantification of fibrosis (lower panel). N =4–7 per group. ( m ) Northern blots and quantification of Anp , Bnp and Serca2a relative to Gapdh . N =4–6 per group. Data are mean±s.e.m. For a – d , f – i , k – m , * P <0.05 versus Ntg, ** P <0.01 versus Ntg, # P <0.05 versus IGF1R, † P <0.05. P values calculated by one-way analysis of variance followed by Fisher least significant difference post hoc pairwise test. For k , § P <0.05 versus Ntg (unpaired t test). GAPDH, glyceraldehyde 3-phosphate dehydrogenase. Full size image IGF1R is protective in HF+AF mice independently of HSP70 Given BGP-15-mediated protection was independent of HSP70 in the HF+AF model ( Fig. 3 ), and IGF1R can increase PI3K-Akt-HSP70 signalling [19] , we deemed it important to examine whether IGF1R was also able to mediate protection in the HF+AF model independently of HSP70. For this purpose, HF+AF-IGF1R-HSP70 KO mice were generated. Hearts from these animals showed deletion of HSP70, increased IGF1R protein expression, with unchanged phosphorylation of Akt ( Fig. 5a ). HF+AF-IGF1R-HSP70 KO mice displayed better cardiac morphology, more favourable chamber dimensions, improved systolic function (fractional shortening) and ECG traces compared with HF+AF-HSP70 KO mice ( Fig. 5b–j , Supplementary Tables 15–17 ). 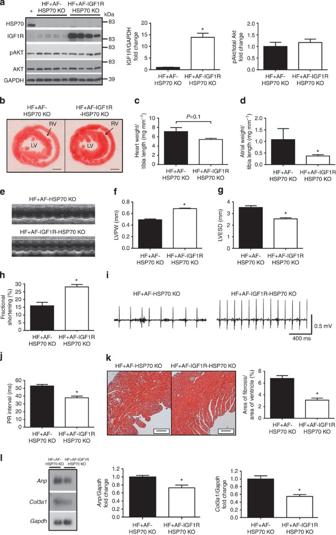Functional improvements in the HF+AF-IGF1R-HSP70 KO mice were associated with less fibrosis, and lower Anp and collagen gene expression ( Fig. 5k,l ). Figure 5: Transgenic overexpression of IGF1R mediates protection in the HF+AF model independently of HSP70. (a) Western blots of HSP70 (deletion of HSP70 in HF+AF-HSP70 KO and HF+AF-IGF1R-HSP70 KO mice), IGF1R, pAkt, total Akt and glyceraldehyde 3-phosphate dehydrogenase (GAPDH), and quantification of IGF1R relative to GAPDH and pAkt relative to total Akt.N=4 per group. ‘+’ represents a heart lysate from a control adult mouse to demonstrate deletion of HSP70 from the HSP70 KO mice. (b) Transverse sections of hearts highlighting the more dilated right and left ventricular chambers (RV and LV) and thinner chamber walls of HF+AF-HSP70 KO in comparison to HF+AF-IGF1R-HSP70 KO. (c,d) Graphs of heart weight/tibia length (TL) and atria weight/TL.N=4 per group. (e) Representative M-mode echocardiograms of HF+AF-HSP70 KO and HF+AF-IGF1R-HSP70 KO mice. (f–h) LV posterior wall thickness (LVPW), LV end systolic dimension (LVESD) and fractional shortening.N=4 per group. (i) ECG traces of HF+AF-HSP70 KO and HF+AF-IGF1R-HSP70 KO mice. (j) PR interval.N=4 per group. (k) LV cross-sections stained with Masson’s trichrome (magnification × 40; scale bar, 200 μm) and quantification of fibrosis.N=4 per group. (l) Northern blots and quantification ofAnpandCol3a1relative toGapdh.N=3–4 per group. Fora,c,d,f–h,j–ldata are mean±s.e.m. *P<0.05 versus HF+AF-HSP70 KO (unpairedt-test). Figure 5: Transgenic overexpression of IGF1R mediates protection in the HF+AF model independently of HSP70. ( a ) Western blots of HSP70 (deletion of HSP70 in HF+AF-HSP70 KO and HF+AF-IGF1R-HSP70 KO mice), IGF1R, pAkt, total Akt and glyceraldehyde 3-phosphate dehydrogenase (GAPDH), and quantification of IGF1R relative to GAPDH and pAkt relative to total Akt. N =4 per group. ‘+’ represents a heart lysate from a control adult mouse to demonstrate deletion of HSP70 from the HSP70 KO mice. ( b ) Transverse sections of hearts highlighting the more dilated right and left ventricular chambers (RV and LV) and thinner chamber walls of HF+AF-HSP70 KO in comparison to HF+AF-IGF1R-HSP70 KO. ( c , d ) Graphs of heart weight/tibia length (TL) and atria weight/TL. N =4 per group. ( e ) Representative M-mode echocardiograms of HF+AF-HSP70 KO and HF+AF-IGF1R-HSP70 KO mice. ( f – h ) LV posterior wall thickness (LVPW), LV end systolic dimension (LVESD) and fractional shortening. N =4 per group. ( i ) ECG traces of HF+AF-HSP70 KO and HF+AF-IGF1R-HSP70 KO mice. ( j ) PR interval. N =4 per group. ( k ) LV cross-sections stained with Masson’s trichrome (magnification × 40; scale bar, 200 μm) and quantification of fibrosis. N =4 per group. ( l ) Northern blots and quantification of Anp and Col3a1 relative to Gapdh . N =3–4 per group. For a , c , d , f – h , j – l data are mean±s.e.m. * P <0.05 versus HF+AF-HSP70 KO (unpaired t -test). Full size image Impact of BGP-15 on membrane fluidity and IGF1R signalling To help understand the association between increased phosphorylation of IGF1R with BGP-15 treatment and potential downstream signalling events, we conducted cell culture experiments, assessed circulating IGF1 levels in mice, performed lipid analyses of atrial tissue, and undertook further protein analyses in ventricular and atrial tissue. First, we examined whether BGP-15 had the potential to enhance the phosphorylation of the IGF1R, as reported for the insulin receptor [12] . For this purpose, neonatal rat ventricular myocytes (NRVMs) were stimulated with IGF1 in the absence and presence of BGP-15 for 48 h. Treatment with IGF1 induced a significant phosphorylation of the IGF1R and this was enhanced in the presence of BGP-15 ( Fig. 6a ). Next, we assessed circulating levels of IGF1 in plasma from a separate cohort of Ntg and HF+AF mice. Cardiac formation of IGF1 increases from the human heart in response to increased haemodynamic load; proposed to act as a protective mechanism [35] . 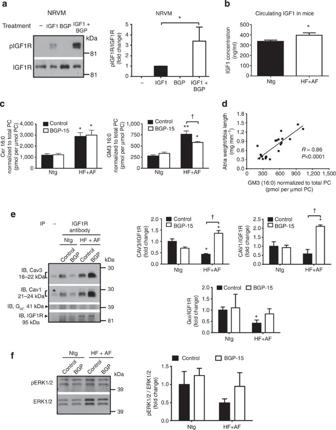It was not technically possible to examine cardiac formation of IGF1 in mice in the current study, however, circulating levels of IGF1 were significantly higher in plasma from HF+AF mice compared with Ntg ( Fig. 6b ). Figure 6: BGP-15 treatment affects IGF1R phosphorylation, ganglioside GM3 levels and content of IGF1R with caveolin-1 and -3. (a) Western blots and quantification of pIGF1R relative to total IGF1R from NRVM without treatment (−), IGF1, BGP-15 or IGF1 with BGP-15 for 48 h. *P<0.05 versus IGF1 alone. Data represent three independent NRVM preparations, with treatments performed in duplicates or triplicates. pIGF1R was undetected in untreated and BGP-15-treated cells, thus IGF1+BGP-15 was normalized to IGF1. *P<0.05 (unpairedt-test). (b) Circulating IGF1 levels in 4.5-month-old Ntg and HF+AF mice. *P<0.05 versus Ntg (unpairedt-test).N=5 for Ntg andN=4 for HF+AF. (c) Quantification of ceramide(16:0) and ganglioside GM3(16:0) in atria from Ntg and HF+AF. *P<0.05 versus Ntg control, **P<0.01 versus Ntg control,†P<0.05.N=5–6 per group. (d) Pearson Correlation between ganglioside GM3 levels and atria weight/tibia length.N=22.P<0.0001. (Pearson correlation). (e) Potential interaction between IGF1R, caveolin-3, caveolin-1 and Gαiin ventricular tissue. Heart lysates were immunoprecipitated with an IGF1R antibody followed by immunoblotting with antibodies for caveolin-3, caveolin-1, Gαi2and IGF1R. Quantification of caveolin-3, caveolin-1 and Gαi2relative to IGF1R. A dash (–) represents a heart lysate with no antibody (negative control); faint signals for caveolin-3, caveolin-1 and Gαi2in the negative control were subtracted from samples incubated with antibody.N=3 per group. *P<0.05 versus Ntg control.†P<0.05. (f) Western blots and quantification of pERK1/2 relative to total ERK1/2 in mouse atria.N=3 for Ntg control and 5–6 for all other groups. Data are mean±s.e.m. Forcande,Pvalues calculated by one-way analysis of variance followed by Fisher least significant differencepost hocpairwise test. IB, immumoblot; PC, phosphatidylcholine. Figure 6: BGP-15 treatment affects IGF1R phosphorylation, ganglioside GM3 levels and content of IGF1R with caveolin-1 and -3. ( a ) Western blots and quantification of pIGF1R relative to total IGF1R from NRVM without treatment (−), IGF1, BGP-15 or IGF1 with BGP-15 for 48 h. * P <0.05 versus IGF1 alone. Data represent three independent NRVM preparations, with treatments performed in duplicates or triplicates. pIGF1R was undetected in untreated and BGP-15-treated cells, thus IGF1+BGP-15 was normalized to IGF1. * P <0.05 (unpaired t -test). ( b ) Circulating IGF1 levels in 4.5-month-old Ntg and HF+AF mice. * P <0.05 versus Ntg (unpaired t -test). N =5 for Ntg and N =4 for HF+AF. ( c ) Quantification of ceramide(16:0) and ganglioside GM3(16:0) in atria from Ntg and HF+AF. * P <0.05 versus Ntg control, ** P <0.01 versus Ntg control, † P <0.05. N =5–6 per group. ( d ) Pearson Correlation between ganglioside GM3 levels and atria weight/tibia length. N =22. P <0.0001. (Pearson correlation). ( e ) Potential interaction between IGF1R, caveolin-3, caveolin-1 and G αi in ventricular tissue. Heart lysates were immunoprecipitated with an IGF1R antibody followed by immunoblotting with antibodies for caveolin-3, caveolin-1, G αi2 and IGF1R. Quantification of caveolin-3, caveolin-1 and G αi2 relative to IGF1R. A dash (–) represents a heart lysate with no antibody (negative control); faint signals for caveolin-3, caveolin-1 and G αi2 in the negative control were subtracted from samples incubated with antibody. N =3 per group. * P <0.05 versus Ntg control. † P <0.05. ( f ) Western blots and quantification of pERK1/2 relative to total ERK1/2 in mouse atria. N =3 for Ntg control and 5–6 for all other groups. Data are mean±s.e.m. For c and e , P values calculated by one-way analysis of variance followed by Fisher least significant difference post hoc pairwise test. IB, immumoblot; PC, phosphatidylcholine. Full size image Work from our group previously demonstrated that BGP-15 activates signalling pathways via enhancing membrane fluidity [34] . In the present study, we assessed membrane fluidity by measuring levels of the G M3 ganglioside (GM3) via lipidomics analysis in mouse atrial samples. Gangliosides are glycosphingolipids, which are abundant in plasma membranes, and increased levels have been implicated in metabolic diseases [36] . GM3 is the main ganglioside in the majority of mammalian cells and is abundant in both the rodent and human heart (representing ≥50% of all gangliosides) [36] , [37] . Levels of ceramide(16:0), a precursor in the synthesis of GM3, were elevated in atria of the HF+AF model compared with Ntg and this was accompanied by an increase in GM3(16:0) ( Fig. 6c ). Treatment with BGP-15 in HF+AF mice was associated with reduced levels of GM3(16:0) in atria compared with HF+AF control ( Fig. 6c ). Furthermore, normalized atrial weight was positively correlated with GM3(16:0) levels ( Fig. 6d ). Caveolae, microdomains of the plasma membrane, are enriched with growth factor receptors including IGF1R, and the interaction between growth factor receptors and caveolin proteins (major components of caveolae) can be disturbed by increased GM3 levels [38] . Owing to inadequate atrial tissue for immunoprecipitation experiments in the current study, the potential interaction between IGF1R and caveolin proteins was assessed in ventricular tissue. The content of caveolin-3 with IGF1R in ventricular tissue was lower in the HF+AF control model compared with Ntg control, and this was enhanced in BGP-15-treated HF+AF mice ( Fig. 6e ). A similar finding was observed for caveolin-1 ( Fig. 6e ). In addition to PI3K-Akt, IGF1R activates other signalling cascades including Ras/Raf-ERK1/2 and G αi (ref. 39 ). The content of G αi with IGF1R was depressed in ventricular tissue from the HF+AF control model compared with Ntg control, but not in the BGP-15-treated HF+AF model ( Fig. 6e ). The phosphorylation of ERK1/2 relative to total ERK1/2 was not significantly altered in atria of the Ntg and HF+AF model ( Fig. 6f ). BGP-15 mediates protection in a second HF and AF mouse model To assess the therapeutic potential of BGP-15 in an independent mouse model with HF and AF, BGP-15 was administered to cardiac-specific muscle-restricted coiled-coil (MURC) Tg mice, which develop DCM, HF and display atrial arrhythmias [40] . MURC activates the Ras homolog gene family, member A (RhoA)/Rho-associated, coiled-coil-containing protein kinase (ROCK) pathway, increases Anp and regulates myofiber organization. MURC mutations are also considered likely causal variants in human DCM; mutations were associated with progressive HF, conduction defects and cardiac arrhythmias [41] . In the MURC model at 3–4 months of age, cardiac morphology and function are less severe than that of the HF+AF model (that is, dnPI3K-Mst1), and episodes of arrhythmia were only identified in approximately 42% of mice at this age [40] . Thus, a cohort of MURC mice and Ntg littermate controls were aged to 11–12 months before treatment with BGP-15 or saline for 4 weeks. BGP-15 had no effect in 11- to 12-month-old Ntg mice ( Supplementary Fig. 8 ). The MURC model was associated with significant atrial enlargement, cardiac dysfunction, arrhythmia, cardiac fibrosis, elevated Anp expression and depressed Serca2a expression ( Fig. 7a–f , Supplementary Tables 18–20 ). BGP-15 treatment improved cardiac outcome and/or attenuated cardiac pathology and molecular abnormalities in the MURC mice ( Fig. 7a–f , Supplementary Tables 18–20 ). Treatment with BGP-15 did not increase HSP70 in atrial tissue of the MURC model, but was associated with an increase in pIGF1R, as observed in the HF+AF model ( Fig. 7g ). pAkt/total Akt was not different between MURC saline and BGP-15-treated mice ( Fig. 7g ). Figure 7: BGP-15 attenuates cardiac pathology and episodes of arrhythmia, and improves cardiac function in the MURC model. ( a ) Representative heart photos from saline and BGP-15-treated Ntg and MURC mice. Scale bar, 2.5 mm. ( b ) Quantification of atria weight/tibia length. * P <0.05 versus Ntg control; † P <0.05. N =3 for Ntg control and 4 for MURC groups. ( c ) Quantification of fractional shortening before and after treatment. * P <0.05, N =4 per group. ( d ) Quantification of the % change in arrhythmia after 4 weeks. * P <0.05 versus Ntg control; † P <0.05. N =3 for Ntg control and 4 for MURC groups. ( e ) LV cross-sections stained with Masson’s trichrome (fibrosis stains blue, magnification × 40; scale bar, 400 μm) and quantification (right panel). * P <0.05 versus Ntg control; † P <0.05. N =3 for Ntg control and 4 for MURC groups. ( f ) Northern blots and quantification of Anp and Serca2a relative to Gapdh . N =3 for Ntg control and 4 for MURC groups. * P <0.05 versus Ntg control; ** P <0.005, *** P <0.001 versus Ntg control; † P <0.05. ( g ) Western blots and quantification of HSP70 relative to GAPDH, pIGF1R relative to total IGF1R and pAkt relative to total Akt in mouse atria. * P <0.05 versus Ntg control. N =3 for Ntg control and 4 for MURC groups. Data are mean±s.e.m. For b , d – g , P values calculated by one-way analysis of variance followed by Fisher least significant difference post hoc pairwise test. For c , P values calculated by paired t -test when comparing the same mice before and after treatment, or one-way analysis of variance followed by Fisher least significant difference post hoc pairwise test. Full size image Here we demonstrate that BGP-15 treatment provided benefit in two independent mouse models with pre-existing HF and arrhythmia. BGP-15 improved cardiac function, reduced episodes of arrhythmia, attenuated atrial enlargement and cardiac fibrosis, and was associated with an improved cardiac molecular profile. We also show that BGP-15-induced protection was associated with an increased phosphorylation of IGF1R, and a potential mechanism of action is via increased membrane fluidity because of reduced ganglioside GM3 levels. In addition, increasing IGF1R in the HF+AF model mimicked the protection observed with BGP-15, and BGP-15 or increased IGF1R provided protection in the HF+AF model independently of PI3K-Akt signalling and HSP70. The majority of studies presented in this report were conducted in the model referred to as ‘HF+AF’ because this model displays a reproducible HF and AF phenotype by 4 months of age, and the age of disease presentation provided a realistic window to study the impact of genetically manipulating HSP70 and IGF1R expression. After establishing that BGP-15 provided benefit in the HF+AF model, later studies were undertaken to examine whether BGP-15 was effective in an unrelated model, which also presents with HF and AF, that is, aged MURC mice. The therapeutic benefit of BGP-15 in the HF+AF model was recapitulated in the MURC model. BGP-15 represented an attractive drug to investigate in a setting of HF and AF because it was previously shown to co-induce HSP70 in skeletal muscle [31] , [32] , and reduced cardiac HSP70 levels were associated with AF in patients [15] , [16] . Furthermore, BGP-15 had been shown to be safe in humans [9] , [10] , [11] , and clinical phase II/b testing for type 2 diabetes has been completed [42] . Interestingly, BGP-15 did not co-induce HSP70 in cardiac muscle of the HF+AF model or the MURC model. Given this unexpected result, a number of experiments were performed in the HF+AF model to demonstrate that BGP-15 was mediating protection independently of HSP70. First, we deleted HSP70 from the HF+AF model, and found that BGP-15 provided cardiac protection in the absence of HSP70. Second, we overexpressed HSP70 in the heart of the HF+AF mouse model, and showed this provided no benefit. To identify potential mechanisms via which BGP-15 may be providing protection in the heart, we explored other known actions of BGP-15. BGP-15 had previously been shown to facilitate the actions of membrane-localized receptor proteins via enhancing membrane fluidity [34] , including increased phosphorylation of the insulin receptor in kidney and adipose cells [12] . Thus, we turned our attention to IGF1R, an insulin receptor family member, which protects the heart in settings of cardiac disease [19] . Phosphorylation of IGF1R was depressed in atrial tissue from the HF+AF model, and was also suppressed in atrial samples from patients with AF. Treatment with BGP-15 in the HF+AF model was associated with higher phosphorylation of IGF1R, and Tg overexpression of IGF1R in the HF+AF model mediated protection, which was comparable to that observed in BGP-15-treated mice. The physiological growth promoting and cardioprotective properties of IGF1R have largely been attributed to the activation of PI3K [19] . However, as the HF+AF mouse model incorporates the dnPI3K transgene (reduces PI3K-Akt signalling by ~80%), we concluded that a PI3K-Akt independent mechanism was largely responsible for BGP-15- and IGF1R-induced protection. Blunted PI3K signalling was confirmed by demonstrating no elevation in the phosphorylation of Akt in hearts expressing the IGF1R transgene. As IGF1R-PI3K-Akt signalling has also been shown to increase HSP70 in the heart [19] , [43] , we generated HF+AF mice with IGF1R overexpressed and HSP70 deleted to confirm that IGF1R could also mediate protection independently of HSP70, as observed for BGP-15. The demonstration that both BGP-15 or increased IGF1R was capable of providing protection in the HF+AF model, independent of the PI3K-Akt pathway and HSP70, is important because signalling via PI3K, Akt and HSP70 is often defective in the aged and/or diseased heart [44] , [45] , [46] , [47] . Previous studies have illustrated that increased IGF1/IGF1R is beneficial in multiple settings of cardiac pathology including DCM, hypertrophic cardiomyopathy (induced by pressure overload) and myocardial infarction [48] . To our knowledge, this is the first study to demonstrate a protective effect of IGF1R on cardiac function and ECG parameters in vivo, which is independent of the PI3K pathway. There is some evidence in vitro to suggest that IGF1R-PI3K-independent pathways can regulate electrical activity in the heart. In neonatal rat cardiac myocytes, IGF1 had an impact on potassium currents that protected myocytes against arrhythmogenesis, and this protection was mediated by both PI3K-dependent and PI3K-independent mechanisms [49] . Identification of drugs that can mediate protection independently of PI3K is of further significance because risk factors for HF and AF including obesity and diabetes have also been associated with impaired PI3K-Akt signalling in the heart [23] , [24] , [25] , [44] . Thus, a therapy that can provide protection independent of PI3K has the potential to be valuable in a number of settings. IGF1R are enriched within caveolae [38] , and previous studies provide support for an interaction between GM3 and the closely related insulin receptor. Phosphorylation of the insulin receptor was enhanced in mice lacking GM3 (ref. 50 ), and insulin receptor signal transduction was attenuated by increased GM3 levels via dissociation of the insulin receptor from caveolae [51] . Based on these data, together with data collected from our in vivo mouse studies, cell culture, lipid and protein analyses, we present a potential mechanism via which BGP-15 treatment may lead to increased phosphorylation of the IGF1R and subsequent cardioprotective signalling ( Fig. 8 ). The HF+AF model is associated with increased atrial GM3 levels, which were positively correlated with atrial weight, suggesting GM3 may contribute to atrial pathology. We propose that increased GM3 levels reduce membrane fluidity, and inhibit phosphorylation of the IGF1R and downstream signalling events via caveolins, which are critical for mediating protection in the healthy heart [52] . Dysregulation of caveolin-1 and caveolin-3 has been associated with cardiac dysfunction in mice [52] , and interestingly a susceptibility locus for AF in humans was located in the caveolin-1 gene ( CAV1 ) [53] . We further hypothesize that in a setting of disease, the heart releases IGF1 as a protective mechanism, and in the presence of BGP-15: GM3 levels are reduced, membrane fluidity is enhanced, phosphorylation of IGF1R is increased and cardioprotective signalling via caveolins is restored ( Fig. 8 ). IGF1R in the heart is recognized to activate multiple pathways involving classic second messengers, phosphorylation cascades, lipid signalling, Ca 2+ transients and gene expression [39] . Furthermore, signalling via IGF1R can occur in multiple subcellular locations, including the plasma membrane, perinuclear T tubules and internalized vesicles. It was not possible to examine all these possibilities in the current study. However, given IGF1R and BGP-15 were not acting via PI3K-Akt signalling, we examined ERK1/2 phosphorylation and the association of G αi2 with IGF1R. Activation of ERK1/2 was not altered by BGP-15 treatment in the HF+AF model. However, the content of G αi2 with IGF1R was significantly lower in ventricular tissue from the HF+AF model but not BGP-15-treated mice. G αi has been shown to associate with IGF1R in other tissue/cell types [54] , [55] , and G αi2 provides protection in the heart [56] , [57] . Thus, this could represent one mechanism by which BGP-15 is mediating protection via IGF1R in the HF+AF model. Figure 8: Schematic representation of BGP-15 protection in a setting of HF and AF. We propose that binding of IGF1R with caveolin-1 and caveolin-3 is important for IGF1R-protective signalling. In the HF+AF model, ganglioside GM3 levels are increased and this disrupts the interaction between IGF1R and caveolins. BGP-15 can restore signalling by attenuating GM3 levels. In the diseased setting, the dotted black line shows the proposed disruption of IGF1R with caveolins because of increased GM3. BGP-15 attenuated GM3 (solid red line) and may attenuate the dissociation between IGF1R and caveolins (dotted red line). In the HF+AF model, PI3K-Akt signalling is blunted (as indicated with a cross, X). The current results suggest IGF1R may mediate protection via Gi, although this will require further investigation. Full size image The current study represents the first demonstration that BGP-15 can improve heart function and reduce episodes of arrhythmia in the mammalian heart in vivo . After commencing the experiments described in this report, it was documented that pre-treatment of Drosophila with BGP-15 was able to protect against tachypacing-induced structural remodelling and contractile dysfunction of the heart [58] . In that study, protection was attributed to increased expression of DmHSP23 (considered to represent a functional orthologue of human HSP27). In the current study, HSP27 levels were elevated in the HF+AF mouse model, but BGP-15 treatment had no additional effect ( Supplementary Fig. 6 ), suggesting that HSP27 is not the mechanism by which BGP-15 attenuates pathology in the mammalian heart. There are limitations to this report, which should be addressed by future studies. First, the efficacy of BGP-15 has currently only been demonstrated in mice with HF and AF. A limitation of using mice to study AF is related to the fast heart rate (HR) and small atrial size in comparison with larger animal models and humans [59] . These features make it necessary to induce AF ex vivo with pacing in most mouse models, and AF is typically not sustained for long periods. The HF+AF mouse model utilized in this study represents one of the few models, which develop AF spontaneously (loss of P waves during periods with irregular RR intervals confirmed using an intracardiac catheter) [20] ; most likely a consequence of the larger atrial size and significant atrial fibrosis compared with other mouse models [20] , [59] . However, the episodic nature of AF in AF mouse models makes exact quantification challenging, and continuous recording with an intracardiac catheter is not possible in a treatment intervention study, as described here. For this reason, we used quantification of the rate of arrhythmia, PR interval and systolic function as a collective readout of disease status. Features of the HF+AF mouse model used in the current study, which have relevance to human HF and AF, include atrial enlargement, atrial and ventricular fibrosis, cardiac dysfunction, progression of disease with age, and dysregulation of genes associated with electrical remodelling [20] . Experiments in larger animal models and a comparison of BGP-15 with other HF drugs (for example, β-blockers, angiotensin-converting enzyme (ACE) inhibitors and angiotensin receptor blockers) could form the basis of future work. Of interest, it was recently reported that β-blocker therapy led to a significant reduction in all-cause mortality in HF patients with sinus rhythm, but not in HF patients with AF [60] . Second, we had limited access to age- and sex-matched samples from patients with and without AF; assessment of pIGF1R should be examined in larger numbers of patients. Third, the current body of work suggests that BGP-15-induced activation of IGF1R could significantly contribute to the protection identified in BGP-15-treated HF+AF mice. However, we cannot directly assess the contribution of IGF1R-mediating protection in the BGP-15-treated HF+AF model. This could theoretically be evaluated by administering BGP-15 to HF+AF-IGF1R KO mice. Although, we consider it highly unlikely this model would be viable given that loss of IGF1R in the heart in another mouse model with defective Akt signalling (mice lacking insulin receptor in the heart) led to death within 17–27 days after birth due to HF [61] . Finally, a more detailed examination of how BGP-15 increases the phosphorylation of IGF1R, signalling downstream of IGF1R, as well as additional mechanisms independent of IGF1R should be conducted in future work. For instance, involvement of caveolae in affecting signalling of receptors is recognized within the field, although the exact functional impact of the interaction has not been clearly outlined, in part because of different methods used to separate caveolae [38] . In the current study, we had insufficient tissue to perform specialized techniques to isolate caveolae and this should be assessed in later work. Furthermore, previous studies have suggested that BGP-15 can protect the heart against ischaemia-reperfusion injury or cardiotoxicity by decreasing reactive oxygen species by modulating poly(ADP-ribose) polymerase, and suppressing JNK and p38 via Akt, respectively [62] , [63] . In summary, mortality associated with HF and AF is significant and the prevalence of these conditions is increasing. Thus, the identification of new therapies is urgently required. The present study has identified BGP-15 as a pharmacological agent with the ability to attenuate pathological atrial and ventricular remodelling, improve heart function and reduce episodes of arrhythmia. We have also discovered a protective role of BGP-15 in the heart, which is mediated independent of HSP70 and PI3K-Akt signalling. As BGP-15 has successfully been administered to humans without serious side effects, this study uncovers a potential novel therapeutic approach for patients with HF and AF. Experimental animals All aspects of animal care and experimentation were approved by the Alfred Medical Research and Education Precinct Animal Ethics Committee. Mice were housed in a 12-h light–dark cycle in a temperature-controlled environment. In this study, we used two models that develop HF over time and display an increased susceptibility to AF: (i) cardiac-specific dnPI3K-Mst1 Tg mice [20] referred to as HF+AF model and (ii) cardiac-specific MURC Tg mice [40] . The HF+AF model displays atrial enlargement and fibrosis, intermittent/episodic AF (confirmed by intracardiac ECG recordings) and systolic dysfunction by 4 months of age [20] . Approximately 42% of MURC Tg show cardiac arrhythmia up to 5 months of age [40] . Thus, for this study, mice were examined at 11–12 months of age; at this age all mice displayed arrhythmia. To assess mechanisms via which BGP-15 had effects in the HF+AF model, the following mice were specifically generated for this study: HF+AF-HSP70 Tg mice, HF+AF-HSP70 KO mice, HF+AF-IGF1R Tg mice and HF+AF-IGF1R-HSP70 KO mice. Generation of genetic mouse models i HF+AF model: male hemizygous cardiac-specific Mst1 Tg mice (C57BL/6, driven by the α myosin heavy chain promoter) [21] were bred with female hemizygous cardiac-specific dnPI3K mice (FVB/N, driven by the α myosin heavy chain promoter) [22] . ii HF+AF-HSP70 Tg mice: male Mst1-dnPI3K mice (HF+AF model, C57BL/6-FVB/N mixed background) were bred with female hemizygous HSP70 Tg mice (overexpression of HSP70 in heart and skeletal muscle utilizing β-actin promoter and a cytomegalovirus enhancer; BALB/c background) [64] . iii HF+AF-HSP70 KO: male Mst1-HSP70 KO mice (C57BL/6 background; HSP70 global KO [65] ) were bred with female dnPI3K-HSP70 KO mice (FVB/N-C57BL/6 background). iv HF+AF-IGF1R Tg mice: male Mst1-dnPI3K (HF+AF model, C57BL/6-FVB/N mixed background) were bred with female hemizygous cardiac-specific IGF1R mice (FVB/N background) [19] . v HF+AF-IGF1R-HSP70 KO mice: male Mst1-dnPI3K-HSP70 KO (C57BL/6-FVB/N mixed background) bred with IGF1R-HSP70 KO mice (FVB/N-C57BL/6 background). All Tgs (Mst1, dnPI3K, IGF1R, HSP70) are hemizygous, and all mice were on the same mixed genetic background for any particular cohort. For (i), (ii), (iv) and (v) littermate controls were used. For (iii), due to the large number of potential combinations of genotypes and small litter sizes, it was not always possible to use littermate controls, but all mice were on the same mixed genetic background and aged matched. Primer sequences for genotyping Tg and KO mouse models are provided in Supplementary Table 21 . Experimental protocols Protocol 1: Adult (~4 month) male HF+AF and Ntg mice were administered with BGP-15 (15 mg kg −1 per day in saline, N-Gene Research Laboratories) for 4 weeks by oral gavage or remained untreated (oral gavage with saline or no gavage). Gavage with saline had no effect on morphological or functional parameters in the HF+AF model ( Supplementary Fig. 3 ). Therefore, untreated mice (no gavage) and mice administered saline are combined and referred to as HF+AF control. Echocardiography and ECG studies were performed before and after treatment. Protocol 2: To determine whether BGP-15 provided protection via HSP70, BGP-15 (15 mg kg −1 per day, oral gavage) was administered to adult (~14 weeks) male and female HF+AF mice deficient for HSP70 (HF+AF-HSP70 KO) for 4 weeks. Protocol 3: To assess whether an increase in HSP70 could mediate protection in the HF+AF model, male HF+AF mice overexpressing HSP70 (HF+AF-HSP70 Tg) were generated and characterized at ~12–13 weeks. Protocol 4: To examine whether overexpression of IGF1R in the heart could provide protection in the HF+AF model, male HF+AF mice overexpressing IGF1R (HF+AF-IGF1R Tg) were generated and characterized at ~16–17 weeks. Protocol 5: To determine whether IGF1R could mediate protection in the HF+AF model independent of HSP70, male and female HF+AF-IGF1R Tg-HSP70 KO mice were generated and characterized at ~11 weeks. Protocol 6: To examine whether BGP-15 had the capacity to provide protection in an additional model with HF and AF, 11- to 12-month-old male MURC Tg were administered with BGP-15 (15 mg kg −1 per day, oral gavage) or saline for 4 weeks. Electrocardiogram ECGs were recorded from anaesthetized mice (1.8% isoflurane) by placing a pair of 27-G needle electrodes subcutaneously (right arm and chest lead equivalent to V5). Signals were sampled for at least 5 min using the Powerlab system and BioAmp (ADInstruments). ECG parameters (PR interval-length of time from the beginning of the P-wave to the beginning of the QRS complex representing atrioventricular conduction, RR interval-interbeat intervals, QRS interval-duration of the QRS complex, P and R-amplitudes, HR) were measured using Chart 5 (ECG analysis module), and arrhythmia (based on a change in HR >30 b.p.m.) was assessed for the entire recording period. As P waves are small in the AF model, PR intervals were also assessed manually by two independent observers. Cardiac structure and function Echocardiography (two-dimensional M-mode) was performed in anaesthetized mice (1.8% isoflurane) using a Philips iE33 ultrasound machine with a 15-MHz linear array transducer. LV wall thicknesses (LV posterior wall; interventricular septum), LV chamber dimensions (LV end-diastolic dimension, LVEDD; LV end-systolic dimension, LVESD) and fractional shortening (FS; [(LVEDD−LVESD)/LVEDD] × 100%) were measured from the short axis of the LV. All measurements were performed with an off-line analysis system (ProSolv Cardiovascular Analyzer 3.5; ProSolv) from at least three beats that were then averaged. Histological analyses Ventricle samples were fixed in 4% paraformaldehyde, dehydrated and embedded in paraffin. Ventricle sections (6 μm) were stained with Masson’s trichrome for quantitative analysis of fibrosis. Percentage fibrosis was calculated by dividing the total area of blue staining (collagen) by the total area of the LV using Image-Pro Plus 6.0. Analysis of human atrial tissue In this study, we performed western blot analysis on previously prepared protein lysates from human atrial tissues, which were collected for a previous study [20] , as well as some additional tissues, which had been stored at −80 °C. Collection of all atrial tissue was approved by the Alfred Hospital (Melbourne) Human Ethics committee, and all patients gave informed consent. Tissue samples of atrial appendages were collected from age-matched male patients undergoing CABG surgery (right appendage only) who did or did not develop acute AF. Medications (statins, β-blockers and ACE inhibitors) were evenly distributed between groups and stopped the night before surgery. Diabetic patients were not included in the study. Further details are provided in Supplementary Table 7 . Protein lysate preparation Hearts were homogenized in 200–300 μl ice-cold Heart Lysis Buffer (1% NP-40, 10% glycerol, 137 mM NaCl, 20 mM Tris–HCl, pH 7.4, 4 μg ml −1 aprotinin 4 μg ml −1 leupeptin, 1 mM phenylmethylsulfonyl fluoride, 4 μg ml −1 pepstatin, 20 mM NaF, 1 mM sodium pyrophosphate, 1 mM orthovanadate, 10 mM EDTA and 1 mM EGTA). Lysates were kept on ice for 15 min before centrifuging at 14,000 r.p.m. for 15 min at 4 °C. Supernatants were collected and protein concentrations were measured using the Bradford method (Bio-Rad). Western blotting Western blotting was performed using 100 μg protein extracted from mouse ventricle, 50 μg from mouse atrial tissue and 70 μg from human atrial tissue. Protein lysates were separated by SDS–polyacrylamide gel electrophoresis, blotted onto polyvinylidene difluoride membrane (Merck) and incubated with primary antibody overnight. The following concentrations of primary antibodies were used: 1:500 phospho-Akt (Cell Signaling, 9271), 1:1,000 Akt (Cell Signaling, 9272), 1:1,000 Hsp70 (Stressgen, 810B), 1:1,000 phospho-IGF-1Rβ (Cell Signaling, 3024), 1:1,000 IGF-1Rβ (Santa Cruz, sc-713), 1:1,000 phospho-Hsp27 (Cell Signaling, 2401), 1:1,000 Hsp27 (Cell Signaling, 2442), 1:5,000 GAPDH (Santa Cruz, sc-32233), 1:200 pERK1/2 (Santa Cruz, sc-7383), 1:1,000 ERK1/2 (Cell Signaling, 9102). Signals were detected by chemiluminescence and quantified using ImageJ 1.44p pixel analysis (US National Institutes of Health). Full immunoblots with molecular weight markers are provided in Supplementary Fig. 9 . Immunoprecipitation Protein lysates (500 μg of protein) were cleared with Protein A Sepharose CL-4B beads (GE Healthcare) in a 50% PBS slurry for 1 h at 4 °C, the beads were pelleted by centrifugation (9,000 g , 1 min at 4 °C) and the cleared supernatant was collected and immunoprecipitated with an IGF1R antibody (10 μl, Santa Cruz, sc-713) overnight at 4 °C. Immunopreciptiates were then coupled to Protein A Sepharose CL-4B beads (GE Healthcare) and washed four times in Heart Lysis Buffer. After the final wash, immunoprecipitates were resuspended in 2 × SDS sample buffer and subjected to SDS–polyacrylamide gel electrophoresis. Immunoblots were then probed with caveolin-1 (1:1,000, BD Biosciences, 610407), caveolin-3 (1:1,000, Santa Cruz, sc-5310), G αi2 (1:1,000, Santa Cruz sc-7276) and IGF1R (1:1,000, Santa Cruz, sc-713). The negative control was a ventricular lysate without addition of antibody. RNA extraction and northern blotting Total RNA was extracted from mouse ventricles using TRI-reagent (Sigma Aldrich). 20 μg of total RNA were separated on a formaldehyde denaturing agarose gel and transferred to a Hybond-N membrane (GE Healthcare) in 20 × saline sodium citrate (SSC) by upward capillary transfer. Membranes were blocked in hybridization solution (50% deionized formamide, 6 × SSC, 5 × Denhardt’s solution, 0.5% SDS) containing 1 mg ml −1 denatured salmon sperm DNA at 42 °C for 1 h before hybridization. Radiolabelled probes ([α- 32 P]dCTP; sequences provided in Supplementary Table 22 ) were prepared using a Prime-a-Gene Labeling System (Promega). Membranes were hybridized with the denatured radiolabelled probes at 42 °C overnight (2 × 10 6 c.p.m. ml −1 of hybridization solution). Membranes were rinsed twice at room temperature (RT) in 2 × SSC, and then washed twice at 42 °C in 2 × SSC/1% SDS for 5 min followed by twice in 0.1 × SSC for 30 min. Amersham Hyperfilm MP autoradiography films (GE Healthcare) were exposed to membranes with an intensifying screen at −80 °C. The correct size of signals was confirmed by the location of the 28S and 18S bands. Full northern blots with 18S and 28S marked positions are in Supplementary Fig. 9 . Reverse transcription–quantitative PCR Complementary DNA was obtained by reverse transcription using a High Capacity cDNA Reverse Transcription Kit (Life Technologies) according to the manufacturer’s recommendations. Reverse transcription–quantitativePCR was performed using TaqMan probes (Life Technologies, Supplementary Table 23 ). Expression was normalized against Hypoxanthine phosphoribosyltransferase 1 ( Hprt1 ) using the 2-ΔΔCt method of quantification. Microarray analysis Kcna5 , Kcnj3 , Gja5 , Gja1 and Cacna1s mRNA expression data were obtained from a previously published microarray data set [20] , deposited in Gene Expression Omnibus of the National Centre for Biotechnology Information database, accession number GSE12420. Lipidomic analysis of atria Atria samples were homogenized and sonicated in 100 μl PBS (pH 7.4). Protein concentration was determined by the Bicinchoninic acid (BCA) protein assay. To each sample (50 μg protein in 10 μl), a mixture of internal standards (1:1, 10 μl) in 200 μl of CHCl 3 /methanol (2:1) was added, then briefly vortexed. Samples were mixed (rotary mixer, 10 min), sonicated (water bath, 30 min at RT) and rested (20 min) at RT. Samples were centrifuged (16,000 g , 10 min) and supernatant was dried under a constant stream of nitrogen gas at 40 °C for approximately 1 h. Extracted lipids were resuspended in 50 μl H 2 O saturated butanol with sonication (10 min), followed by 50 μl of 10 mM NH 4 COOH in methanol. Extracts were centrifuged (3,350 g , 5 min), and the supernatant stored in glass vials with Teflon insert caps at −80 °C until required. Lipid analysis was performed on lipid extracts (5 μl; sonicated in a water bath for 30 min at RT before use) by liquid chromatography electrospray ionization tandem mass spectrometry using an Agilent 1,200 liquid chromatography system and an Applied Biosystems API 4,000 Q/TRAP mass spectrometer with a turbo-ionspray source (350 °C) [66] , [67] . Data were analysed in Multiquant 2.1 software and specific lipid species normalized to total phosphatidylcholine levels. Cell culture Primary cultures of NRVM were prepared from 1- to 3-day-old Sprague–Dawley strain rats. Ventricles from 1- to 3-day-old Sprague–Dawley rats were minced, trypsinized overnight at 4 °C and ventricular cells isolated by six subsequent collagenase digestion steps at 37 °C. Non-cardiac myocytes were separated from the cardiac myocytes by differential preplating. Cardiac myocytes were then plated on 10 cm 2 culture dishes (Thermo Scientific) at 5 × 10 4 cells cm −2 , giving a confluent monolayer of spontaneously contracting cells after 24 h. The cells were maintained at 37 °C and 5% CO 2 in culture medium of Dulbecco’s modified Eagle’s medium, supplemented with 10% (v/v) fetal bovine serum, 9.0 g l −1 D -glucose, 4 mM L -glutamine and penicillin/streptomycin (100 units ml −1 ). The serum was removed after 48 h, and cells starved for 24 h before experimental treatment. NRVMs were treated with IGF1 alone (10 nM, Novozymes Biopharma AU Ltd, #CM001, made at a concentration of 1 mg ml −1 in 10 mM HCl before dilution in media on the day of the experiment), BGP-15 alone (50 μM, N-Gene, made up in saline) or IGF1 (10 nM) with BGP-15 (50 μM) for 48 h. Cells were collected for subsequent protein analysis by western blotting. IGF1 assay Blood was collected by cardiac puncture from a small cohort of anaesthetized (pentobarbitone, 80 mg kg −1 , i.p.) HF+AF and Ntg mice. IGF1 in plasma was measured using a Mouse/Rat IGF-1 Immunoassay Quantikine ELISA Kit (R&D Systems Inc., MG100). Study design, sample size, randomization and exclusion criteria The main objective of this study was to assess the impact of BGP-15 on cardiac function and conduction in a mouse model, which displays AF and develops HF over time. Sample sizes were initially estimated based on defining differences in morphology (for example, atrial weight), ECG parameters and cardiac function from the original characterization of the AF model [20] . Mice were randomized to BGP-15 treatment and control groups. Echocardiography and ECG studies were performed blinded. In the initial experimental design, all mice were to be characterized at approximately 5 months of age after treatment and/or functional assessment. However, the HF+AF-HSP70 KO model did not tolerate gavage well at 4 months of age, and some of the other genetic models died before 5 months of age (observed during the initial generation of mice, before any studies). Thus, the end point of these studies was revised. Importantly, all mice within the same cohorts are age matched. Male mice were used for the majority of studies to eliminate any impact of gender. However, this was not possible for two cohorts because of the large number of potential combinations of genotypes (HF+AF-HSP70 KO: protocol 2 and HF+AF-IGF1R Tg-HSP70 KO: protocol 5). In these cohorts, no significant gender differences were observed based on morphology, function or signalling. One 11- to 12-month-old Ntg mouse from the MURC Tg cohort was excluded because a large tumour (>1 g) was identified at autopsy and the potential impact of this tumour was unknown. For some mice, it was not possible to obtain accurate ECG or echocardiography parameters before or after treatment (for example, noisy ECG traces because of electrical interference). In this instance, traces/images were removed in a blinded manner before measurement and statistical analyses. Assessment of fibrosis and collection of ECG parameters were automated or performed blinded for manual measures, for example, PR interval. Statistics Results are presented as mean±s.e.m. For statistical analyses and graphs, we used StatView and GraphPad Prism software v.6.02. Differences between groups were identified using one-way analysis of variance followed by Fisher least significant difference post hoc pairwise tests (when the ANOVA was significant). All pairwise P values are two-sided. Unpaired t -tests were used when comparing two groups for a single measure, and paired t -tests were used when comparing the same mice before and after treatment for a single measure. A value of P <0.05 was considered significant. All relative units are expressed as a fold change with the relevant control group normalized to 1. How to cite this article: Sapra, G. et al. The small-molecule BGP-15 protects against heart failure and atrial fibrillation in mice. Nat. Commun. 5:5705 doi: 10.1038/ncomms6705 (2014).